Strikingly distinctive NH3-SCR behavior over Cu-SSZ-13 in the presence of NO2 Commercial Cu-exchanged small-pore SSZ-13 (Cu-SSZ-13) zeolite catalysts are highly active for the standard selective catalytic reduction (SCR) of NO with NH 3 . However, their activity is unexpectedly inhibited in the presence of NO 2 at low temperatures. This is strikingly distinct from the NO 2 -accelerated NO x conversion over other typical SCR catalyst systems. Here, we combine kinetic experiments, in situ X-ray absorption spectroscopy, and density functional theory (DFT) calculations to obtain direct evidence that under reaction conditions, strong oxidation by NO 2 forces Cu ions to exist mainly as Cu II species (fw-Cu 2+ and NH 3 -solvated Cu II with high CNs), which impedes the mobility of Cu species. The SCR reaction occurring at these Cu II sites with weak mobility shows a higher energy barrier than that of the standard SCR reaction on dynamic binuclear sites. Moreover, the NO 2 -involved SCR reaction tends to occur at the Brønsted acid sites (BASs) rather than the Cu II sites. This work clearly explains the strikingly distinctive selective catalytic behavior in this zeolite system. Increasingly stringent mobile source emission regulations have been pursued around the world to tackle environmental pollution. Nitrogen oxides (NO x ) are inevitable gaseous pollutants emitted from internal combustion engines. Selective catalytic reduction of NO x with NH 3 (NH 3 -SCR) is the most widely adopted technology for the removal of NO x from diesel engines [1] , [2] . The successful commercialization of Cu-SSZ-13 as an NH 3 -SCR catalyst is a significant achievement for diesel engine exhaust post treatment [3] . In the past decade, numerous studies have endeavored to uncover the standard SCR (SSCR) reaction mechanism [4] , [5] , [6] , [7] , hydrothermal deactivation mechanism [8] , [9] , [10] , [11] , and SO 2 poisoning deactivation mechanism [12] , [13] , [14] , and to develop economic and sustainable synthesis methods for Cu-SSZ-13 [15] , [16] , [17] , [18] , bringing about continuous optimization of Cu-SSZ-13 for commercial SCR catalysts. In actual application, a diesel oxidation catalyst (DOC) is utilized to oxidize carbon monoxide (CO) and hydrocarbons (HCs), accompanied by partial oxidation of NO to NO 2 . The formed NO 2 can participate in the NH 3 -SCR process through the so-called “fast SCR” reaction (FSCR, reaction 1, consisting of reactions 2 and 3). It is generally believed that the deNO x efficiency of the FSCR reaction should be higher than that of SSCR (reaction 4) due to bypassing the oxidation of NO, which is usually the rate-limiting step in the SSCR reaction on V-based and Fe-zeolite catalysts [19] , [20] . NO+NO_2+2NH_3→ 2N_2+3H_2O
 (1) 
    2NO_2+2NH_3→ NH_4NO_3+N_2+H_2O
 (2) 
    NO+NH_4NO_3→N_2+NO_2+2H_2O
 (3) 
    4NO+4NH_3+O_2→ 4N_2+6H_2O
 (4) However, there have been few studies reporting that NO 2 measurably promotes the NH 3 -SCR efficiency over Cu-SSZ-13 catalytic systems. On the contrary, inhibition of NO conversion by NO 2 was found over Al-rich Cu-SSZ-13 catalysts due to NH 4 NO 3 formation, which is the so-called “abnormal fast NH 3 -SCR reaction” [21] . In our recent study, we found that the inhibiting effect of NO 2 was closely related to Brønsted acid sites (BASs) and can be alleviated by hydrothermal aging due to the decrease in the number of BASs in Cu-SSZ-13 [22] . Therefore, we speculated that NO 2 reduction probably occurs at BASs. Also, we previously observed the reaction between NO and NH 4 NO 3 occurring at BASs over the H-SSZ-13 catalyst [23] . Furthermore, Kubota et al. found that NO reacts with NH 4 NO 3 more rapidly than NH 4 NO 3 decomposition over H-AFX and H-CHA zeolites [24] , [25] . However, the situation in Cu-containing zeolites is more complicated. McEwen et al. found that four-fold-coordinated Cu(II) species dominate the Cu-SSZ-13 catalyst under FSCR conditions, which differs from the composition under SSCR conditions, where Cu(I) and Cu(II) species both exist [26] . Paolucci et al. investigated the oxidation process of Cu(I)(NH 3 ) 2 species by O 2 and NO 2 . It was found that oxidation by NO 2 occurred at isolated Cu sites, rather than at the Cu dimer sites required for O 2 activation [5] . More recently, Liu et al. investigated the FSCR mechanism over the Cu-OH site on Cu-CHA zeolite and showed the important role of BASs in the FSCR reaction [27] . Therefore, it can be concluded that the FSCR reaction pathway over Cu-SSZ-13 is unique and different from other catalytic systems where NO 2 accelerates SCR rates. The active sites as well as redox pathways may change over Cu-SSZ-13 in the presence of NO 2 . Compared to the relatively few studies on the FSCR reaction mechanism, researchers have conducted numerous experimental and theoretical studies to explore the SSCR reaction mechanism in the past decade. Thus, the SSCR mechanism has been relatively clear, in which dynamic binuclear Cu + species are the primary active sites [4] , [5] , [28] . However, the influence of NO 2 on the active Cu sites and the mechanism of the NO 2 -involved SCR reaction are barely discussed, and are worth exploring since NO and NO 2 always coexist in actual applications. In this study, the SCR reaction over the Cu-SSZ-13 catalyst in the presence of both NO and NO 2 was studied by kinetic measurements. In situ X-ray absorption fine structure (XAFS) measurements were applied to reveal the state of copper species under SSCR (with only NO as NO x ), FSCR (equal mixture of NO and NO 2 as NO x ) and NO 2 -SCR (only NO 2 as NO x ) reaction conditions. Density functional theory (DFT) calculations were conducted to identify the NO 2 -involved SCR reaction pathways. These results provide new insights into the role of NO 2 in the NH 3 -SCR reaction and shed light on the actual application of Cu-SSZ-13 catalysts in the presence of both NO and NO 2 . Kinetic studies of NO x conversion under SSCR, FSCR and NO 2 -SCR conditions We first carried out kinetic studies on the SSCR reaction, with the results shown in Fig. 1 and Supplementary Fig. 1 . The SSCR rate increases linearly with the square of Cu loading when the Cu loading is below 1.7 wt.% (magnified in Fig. 1b ), indicating the participation of Cu pairs in the standard NH 3 -SCR reaction. Previous studies have reported that Cu I dimers are formed with O 2 activation in the oxidation half-cycle (Cu I →Cu II ) [4] , [5] . Recently, Hu et al. also proposed a Cu II -pair-mediated low-temperature reduction half-cycle (Cu II →Cu I ) [6] . Chen et al. also indicated the participation of Cu pairs in the reduction half-cycle [29] . Therefore, the formation of a Cu pair in the same cage is significantly important for the overall standard NH 3 -SCR reaction process. The increase trend slows down with further rise in the Cu loading. The turnover frequency (TOF) shows a volcano-type tendency, with a maximum at Cu loading of 1.7 wt.% (Fig. 1c ). The increase in TOF at low Cu loading is attributed to the quadratic increase in the SSCR rate. At high Cu loading, however, the decline of TOF is probably due to the underutilization of the active Cu sites. According to the calculation method reported by Jones et al. [30] , every 2.4 and 3.5 CHA cages contain one Cu ion for Cu 3.8 -SSZ-13 and Cu 2.6 -SSZ-13 samples, respectively. The formed Cu-NH 3 complex or dimer Cu species under SSCR conditions probably impede the access of reactants to the Cu ions deep inside the pores, causing inefficiency in the use of Cu ions [31] . The activation energy (Ea) and pre-exponential factor (A) both increase with the increase in Cu loading, which was also observed by Gao et al [31] . Recently, Krisha et al. reported that the Ea of Cu I oxidation increased monotonically with Cu density in a fixed kinetic regime due to the non-mean-field behavior of Cu-SSZ-13 in the NH 3 -SCR reaction and that the Ea of Cu II reduction was unchanged when the Cu load was higher than 0.69 wt.% [32] . On the other hand, the kinetic relevance of Cu II reduction increased with increasing Cu ion density, the Ea of which was higher than that of Cu I oxidation [30] , [32] . Therefore, the increase of the Ea in Cu I oxidation and kinetic relevance of Cu II reduction both contributed to the increase in the Ea of the SSCR reaction. Fig. 1: Kinetic analysis of standard SCR reaction. a SSCR reaction rates as a function of Cu loading. b SSCR reaction rates as a function of the square of Cu loading. c SSCR turnover frequencies (TOF) as a function of Cu loading. d Activation energies (Ea) and pre-exponential factors (A) with different Cu loadings. Full size image Then, the FSCR reaction over Cu-SSZ-13 was carried out as shown in Supplementary Figs. 2a and 3a . Compared to the SSCR reaction, the NO x conversion over Cu3.8-SSZ-13 was significantly inhibited in the presence of NO 2 , which was strikingly distinct from the NO 2 -accelerated NO x conversion over Fe-based zeolite and oxide catalysts (Supplementary Fig. 3 ). Supplementary Fig. 2 shows the NO x , NO and NO 2 conversion levels over Cu-SSZ-13 with different Cu loadings under steady-state FSCR conditions. We normalized the NO and NO 2 reaction rates by the catalyst weight as a function of Cu loading, with the results shown in Fig. 2a , b, respectively. The NO consumption rates under FSCR and SSCR condition were compared (Supplementary Fig. 4 ) and the result showed that NO reduction was severely suppressed at low temperatures under FSCR conditions. The extremely low NO conversion at low temperatures was previously thought to be resulted from zeolite pore blocking by the formation of stable NH 4 NO 3 [21] , [23] . The NH 4 NO 3 formation was verified by the observation of N 2 O in an FSCR-TPD experiment (Supplementary Fig. 5 ), since the N 2 O mainly originated from NH 4 NO 3 decomposition. Interestingly, the NO 2 reduction markedly decreased with the increase in Cu loading, while it increased as the number of BASs rose at low temperatures (Fig. 2b, c and Supplementary Fig. 6 ). This demonstrated that the block of active sites by NH 4 NO 3 was not the only reason for the NO 2 -inhibition effects, otherwise both NO and NO 2 reduction were inhibited. The BASs primarily participated in the reduction of NO 2 , which was also observed in the NO 2 -SCR reaction (Supplementary Fig. 7 ). Moreover, the turnover frequency (TOF) of NO 2 on BASs hardly changed as the number of BAS varied. Supplementary Fig. 8 presents the NO 2 reaction rate as a function of Cu loading and BASs under NO 2 -SCR conditions, which showed the same trend as that in the co-existence of NO and NO 2 . Moreover, we carried out the NO 2 -SCR reaction over H-SSZ-13 and Cu 2.6 -SSZ-13 with different Si/Al ratios and found that the zeolites with low Si/Al exhibited high NO x conversion due to their high numbers of BASs at low temperatures (Supplementary Fig. 9 ). The above results indicated that NO 2 primarily reacted at BASs while NO was difficult to be reduced in the presence of NO 2 . NO 2 disproportionation occurs on the BASs to form nitrates and adsorbed NO + , which then react with NH 3 to form NH 4 NO 3 and NH 2 NO, respectively [33] , [34] , [35] . It is generally known that NO can be effectively reduced at Cu sites. However, the formation of NH 4 NO 3 impedes NO access to the active Cu sites. Instead, NO reacts with NH 4 NO 3 at BASs to form N 2 and NO 2 through reaction (3) (TPSR shown in Supplementary Fig. 10 ). Furthermore, the NO and NO 2 conversion levels over Cu2.6-SSZ-13 and Cu0.4-SSZ-13 under SSCR, FSCR and NO 2 -SCR conditions are separately depicted in Supplementary Fig. 11 . For Cu2.6-SSZ-13 sample, the NO conversion under SSCR conditions was remarkably higher than that under FSCR conditions, which indicated that the SSCR reaction pathway was significantly inhibited under FSCR conditions. We ascribed the low NO conversion to the reaction with NH 4 NO 3 (i.e., FSCR reaction) and the extra NO 2 conversion to the reaction between NO 2 and NH 3 . For Cu0.4-SSZ-13 sample, the NO conversion under FSCR conditions was likewise inhibited compared to that under SSCR conditions. Differently, the NO 2 conversion under FSCR and NO 2 -SCR conditions were relatively higher than the NO conversion under SSCR conditions due to the insufficient Cu active sites for SSCR reaction. As a result, the FSCR rates of NO x can also be higher than SSCR rates of NO x especially when the Cu-zeolite behaves low NO conversion (low Cu loadings, hydrothermal aging state, etc. ), which was observed in previous studies [23] , [27] , [36] , [37] . In another word, the NO conversion was inhibited in the presence of NO 2 , while the effect of NO 2 on NO x conversion was uncertain and relates to NO 2 conversion under FSCR conditions as well as NO x conversion under SSCR conditions. Fig. 2: Kinetic analysis of fast SCR reaction. a NO reaction rates as a function of Cu loading over Cu-SSZ-13 catalysts in NO and NO 2 gas mixtures. b NO 2 reaction rates as a function of Cu loading over Cu-SSZ-13 in NO and NO 2 gas mixtures. c NO 2 reaction rates as a function of BASs over Cu-SSZ-13 in NO and NO 2 gas mixtures. d NO 2 turnover frequencies (TOFs) as a function of BASs in NO and NO 2 gas mixtures. Full size image Wavelet transform analysis of in situ EXAFS measurements Further, we conducted in situ XAFS measurements on Cu-SSZ-13 samples to uncover the valence state and coordination of copper species under different conditions. Wavelet transform (WT) analysis of extended X-ray absorption fine structure (EXAFS) spectra is a powerful technique to resolve overlapping contributions from different neighbor atoms at close distances around the absorber. As shown in Fig. 3a , the pretreated sample shows a distinct first shell peak at (4.5 Å -1 , 1.3 Å), which is associated with contributions from framework oxygen atoms. This result suggested that the copper species mainly exist as fw-Cu 2+ species, which have high coordination numbers [28] . For the second shell sphere (R(Å) > 2 Å), two lobes, at (3.5 Å −1 ,2.8 Å) and (6.5 Å −1 3.3 Å), are well-resolved due to the different backscattering properties of various atoms, which strongly depend on the atomic number. The first lobe is assigned to the second-shell oxygen atom due to the low k value of oxygen atoms. The latter one is attributed to the signals from the Si or Al atoms of the framework. Although some studies attributed the latter lobe to the Cu-Cu contributions in oxygen-bridged Cu dimers [38] , [39] , we scarcely observed CuO x species in X-ray absorption near edge structure (XANES) and EXAFS profiles (Supplementary Fig. 12 ) and did not carry out the procedure of introducing O 2 to NH 3 -treated Cu-SSZ-13 to form oxygen-bridged Cu dimers with four NH 3 ligands. Therefore, we deduced that the lobe at 6.5 Å −1 is primarily derived from the framework Si or Al atoms in the second shell in this work. In fact, the copper species in Cu-SSZ-13 are initially in the solvated state as [Cu(H 2 O)n] 2+ under ambient conditions, which weakens the interaction between copper species and the zeolite framework [28] , [40] . High-temperature treatment in O 2 /N 2 removes the coordinated water molecules and oxidizes copper species to Cu 2+ . As a result, the copper species are in a high valence state and strongly interact with the zeolite framework through electrostatic forces. Fig. 3: WT plots for EXAFS spectra of Cu-SSZ-13 treated under different conditions at 200 °C. a Cu-SSZ-13 pretreated in O 2 /He. b NO adsorption. c NH 3 adsorption. d NO + NH 3 adsorption. e NO + NH 3 co-adsorption followed by reaction with O 2 . f NO + NH 3 co-adsorption followed by reaction with NO 2 . g SSCR conditions. h FSCR conditions. i NO 2 -SCR conditions. Full size image After NO adsorption, Cu 2+ ions are partially reduced, resulting in a slight decrease in the coordination numbers (CNs) of the first shell, denoted by the decrease and weakening of the colored area (Fig. 3b ). The lobes resulting from the contributions of the second shell stretched to (3.5 Å −1 , 3.1 Å) and (6.5 Å −1 , 3.7 Å), respectively. When the pretreated sample was exposed to an NH 3 or NO + NH 3 atmosphere, the signal of the first shell sharply decreased (Fig. 3c, d ), suggesting that the CNs of the Cu ions significantly declined due to their reduction. Moreover, the two lobes are not well-resolved in the spectra, indicating a decrease in the scattering from the second shell. This is consistent with the formation of dynamic [Cu(NH 3 ) 2 ] + species, which is supported by the appearance of feature B in Supplementary Fig. 13a after NH 3 or NO + NH 3 adsorption. After oxidation by O 2 and NO 2 , the CNs of the first shell increased to a level similar to that of the pretreated sample, accompanied by the formation of two well-resolved lobes at the second shell (Fig. 3e, f ). This demonstrated that Cu(NH 3 ) 2 + species are oxidized into Cu II ions and that the interaction between the Cu 2+ ions and the zeolite framework is recovered. Besides the scattering by framework Si (or Al), the second lobe at 6.5 Å −1 probably resulted from the scattering of the second shell Cu species, since oxygen-bridged Cu dimers are formed after Cu I (NH 3 ) 2 oxidation by O 2 [5] , [38] . Compared with oxidation by O 2 , oxidation by NO 2 resulted in a higher signal for the lobe at ~6.5 Å −1 , indicating that more Cu I species are oxidized into Cu II ions (fw-Cu II or NH 3 -solvated Cu II species with high CNs) during the reaction with NO 2 . This phenomenon is consistent with the result reported by Paolucci et al. showing that NO 2 can oxidize the residual Cu I (NH 3 ) 2 species that cannot be oxidized by O 2 . As also reported by Paolucci, the transient oxidation of Cu I (NH 3 ) 2 species by NO 2 is a single-site process without formation of Cu dimers. Therefore, it can be inferred that the presence of NO 2 probably changed the SCR reaction active sites from dimer Cu to isolated Cu species, which further influence the SSCR reaction. This deduction indicated that most Cu species are bonded with the zeolite framework and that the mobility of Cu species is limited during the process of Cu I (NH 3 ) 2 oxidation by NO 2 . Although the transient reaction can reflect the Cu state and coordination during half-cycles, it was deemed more meaningful to identify the Cu species under FSCR reaction conditions. Figures 4g–i depicts 2D plots of the WT EXAFS spectra under SSCR, FSCR and NO 2 -SCR conditions. Under SSCR conditions, the WT EXAFS spectra resemble the ones in Fig. 3c, d . The first shell peak weakened under SSCR conditions, indicating a decrease in the CNs of Cu species. The absence of the lobes at the second shell suggests the easy mobility of the copper complex due to the NH 3 solvation effect. In the presence of NO 2 , however, the CNs of the first shell significantly increased, indicating the oxidation of copper species, which was also supported by the results of McEwen et al. [26] . Moreover, two well-resolved lobes at the second shell are observed, suggesting that oxidization leads to the copper species becoming closely coordinated with the zeolite framework, which limits their mobility during the SCR reaction. The WT EXAFS spectra are consistent with the Fourier-transformed (FT) EXAFS results (Supplementary Fig. 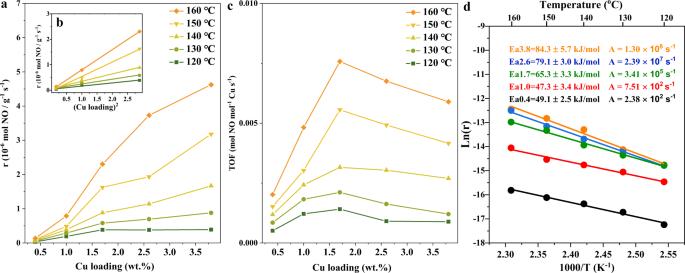Fig. 1: Kinetic analysis of standard SCR reaction. aSSCR reaction rates as a function of Cu loading.bSSCR reaction rates as a function of the square of Cu loading.cSSCR turnover frequencies (TOF) as a function of Cu loading.dActivation energies (Ea) and pre-exponential factors (A) with different Cu loadings. 14 and Table 1 ), which are discussed in detail in the Supporting Information. The above results proved the existence of greater amounts of dynamic Cu I (NH 3 ) 2 species under SSCR reaction conditions than that under FSCR and NO 2 -SCR reaction conditions. Notably, although we proved the existence of significant framework-bound Cu II species under FSCR conditions, the NH 3 -solvated Cu II species cannot be ruled out by the XAFS experiment. Indeed, the NH 3 -solvated Cu II species existed, as indicated by the observation of NH 3 desorption from Cu sites in FSCR-TPD profiles (Supplementary Fig. 5 ), which was consistent with the computed phase diagram reported by Paolucci et al. [28] . Therefore, we next turned to the DFT calculation to investigate the possible FSCR reaction pathways over fw- and NH 3 -solvated Cu II [Cu 2+ and (Cu II OH) + ] species, BASs and dimer Cu species. Fig. 4: Reaction pathway of the fast SCR cycle at Z 2 Cu II site. a Gibbs free energy profile. b Optimized geometries of the reactants, transition states (TSs) and products for all elementary steps are presented in the lower panel. Except for the O atoms linked to the Cu 2+ ion, all other atoms of the zeolite framework are omitted for clarity. Orange, red, blue and white circles denote Cu, O, N and H atoms, respectively. Full size image DFT calculation We first calculated the FSCR reaction pathway over fw-Cu II species (Fig. 4 ). The framework-bound Cu II first adsorbs two NH 3 molecules without separation from the framework, which then interacts with NO 2 to form Z 2 Cu II NH 3 OH and NH 2 NO species (B → C). The Z 2 Cu II NH 3 OH further adsorbs an NH 3 molecule and reacts with NO, resulting in the formation of Z 2 Cu II NH 3 , NH 2 NO and H 2 O (E → F), which was predicted to be the rate-determining step of the SCR reaction cycle with a high energy barrier of 1.92 eV. The formed NH 2 NO is easily decomposed into N 2 and H 2 O through a series of H-migration and isomerization processes (Supplementary Fig. 16 ) [29] . Last, the gaseous NH 3 molecules are supplied to regenerate the initial A species. Next, the FSCR reaction pathway over ZCu II OH was calculated and depicted in Fig. 5 . ZCu II OH first adsorbs an NH 3 molecule to reach a coordinatively saturated state, which interacts with NO 2 to form an HNO 3 molecule without any energy barrier. The B species is actually considered to be NH 4 NO 3 adsorbed on Cu sites. Next, the adsorbed HNO 3 reacts with NO from the gas phase with an energy barrier of 0.87 eV, resulting in the formation of adsorbed HNO 2 and the release of an NO 2 molecule (C → D). Then, the adsorbed HNO 2 reacts with the NH 3 ligand to generate NH 2 NO and H 2 O. As the desorption of N 2 and H 2 O molecules occurs, NH 3 and NO 2 are adsorbed at the Cu site and react to generate NH 2 NO and -OH groups. With the decomposition of NH 2 NO into N 2 and H 2 O, the ZCu II OH site is regenerated. The rate-determining step of the FSCR cycle over the ZCu II OH site corresponds to the reaction of adsorbed HNO 2 with an NH 3 ligand to produce NH 2 NO and H 2 O (E → F), with an energy barrier of 1.58 eV. Fig. 5: Reaction pathway of the fast SCR cycle at ZCu II OH site. a Gibbs free energy profile. b Optimized geometries of the reactants, TSs and products for all elementary steps are presented in the lower panel. Except for the two O atoms linked to the Cu-OH group, all other atoms of the zeolite framework are omitted for clarity. All legends are the same as those in Fig. 4 . Full size image In addition, the FSCR reaction pathways over NH 3 -solvated Cu II species [Cu II and (Cu II OH) + ] were also calculated and presented in Supplementary Fig. 17 , 18 . All the energy barriers were found to be relatively high (1.54 and 1.65 eV). Moreover, we consider the possibility that various NH 3 -solvated Cu II species diffuse into an adjacent cage to form Cu II -pairs as shown in Supplementary Fig. S15 . As expected, the formation of Cu II pairs from Cu II (NH 3 ) 4 and Cu II NO 2 (NH 3 ) 3 is both thermodynamically and kinetically inhibited due to the steric effect as well as strong interaction with zeolite framework. However, it should be noted that Cu II OH(NH 3 ) 3 is different from the other forms since binuclear Cu II OH(NH 3 ) 3 in one cage is thermodynamically more stable than the isolated configuration. Villamaina et al. validated the formation of Cu II (OH)(NH 3 ) x dimeric complexes in the oxidation atmosphere through CO + NH 3 titration experiment [41] . Hu et al. proposed that Cu II (OH)(NH 3 ), which is structurally similar to Cu I (NH 3 ) 2 + that has one charge and two ligands, acts as inter-cage transportation medium [6] . The Z2Cu II species can transform ZCu II (OH) by NH 3 -assisted hydrolysis to achieve the Cu pairing [42] . However, the regeneration of Cu II (OH) in dimeric form showed a high energy barrier of 1.58 eV (A → B in Supplementary Fig. S19 ), suggesting that the dimeric Cu II (OH) species were not highly active in the FSCR reaction. The FSCR reaction pathway at BASs is displayed in Fig. 6 . NH 3 is adsorbed on the BASs to form NH 4 + species. Two NO 2 molecules interact with the NH 4 + species to form NH 4 NO 3 species and release an NO molecule without any energy barrier (A → B). The release of NO was also observed in our previous studies during NO 2 adsorption on H-SSZ-13 zeolite [43] . Then, NO interacts with an NH 3 from the gas phase to form an NH 3 ∙ ∙ ∙ NO complex, which further reacts with NH 4 NO 3 to form NH 4 + , HNO 3 , and NH 2 NO via an H-migration process (B → C). NH 2 NO is decomposed into N 2 and H 2 O. Subsequently, HNO 3 reacts with NO from the gas phase, resulting in the formation of HNO 2 and the release of an NO 2 molecule (E → F). Reaction between HNO 2 and NH 4 + species leads to the formation of an NH 3 ∙ ∙ ∙ NO complex and an H 2 O molecule. The NH 3 ∙ ∙ ∙ NO complex transfers an H atom to regenerate the BAS and changes into NH 2 NO, which then decomposes into N 2 and H 2 O. The whole catalytic cycle is completed. The overall energy barrier of the FSCR over the Brønsted acid site is 1.27 eV, which corresponds to the reaction between NH 4 NO 3 and the NH 3 ∙ ∙ ∙ NO complex, much lower than that over various Cu sites. The DFT-calculated results indicate that the FSCR process in the SSZ-13 zeolite system tends to occur at BASs. Fig. 6: Reaction pathway of the fast SCR cycle at BAS. a Gibbs free energy profile. b Optimized geometries of the reactants, TSs and products for all elementary steps. Except for the Si and Al atoms linked to the OH group, all other atoms of the zeolite framework are omitted for clarity. Yellow and pink circles denote Si and Al atoms, respectively. All other legends are the same as those in Fig. 4 . Full size image In summary, by combining the analysis of in situ spectroscopic measurements with DFT calculations, we found that NO 2 leads to the deep oxidation of copper species as Cu II species (fw-Cu II and NH 3 -solvated Cu II with high CNs), which significantly inhibits the mobility of Cu sites. As a result, the FSCR reaction occurs primarily at the BASs even though it has a higher energy barrier (1.27 eV) than the locally homogeneous SSCR reaction at dynamic sites (about 1.0 eV). This work reveals the origin of the abnormal NH 3 -SCR behavior over the commercial Cu-SSZ-13 catalyst in the presence of NO 2 . Sample preparation The initial Cu-SSZ-13 zeolite was in situ synthesized by a one-pot method [15] . The ratio of Na 2 O/Al 2 O 3 /H 2 O/SiO 2 /Cu-TEPA was 3.5/1.0/200/25/3 and the crystallization of the zeolite was performed at 120 °C for 5 days. Due to the excess Cu in the initial product, aftertreatments were required to optimize the Cu contents and distribution. In detail, the as-synthesized Cu-SSZ-13 was post-treated with 0.1 mol/L HNO 3 at 80 °C for 12 h to remove CuO x species. After calcination at 600 °C, the sample was stirred in NH 4 NO 3 solution (0.01~0.2 mol/L) at 40 °C for the second post-treatment process, followed by filtration, washing, drying and calcination at 600 °C. 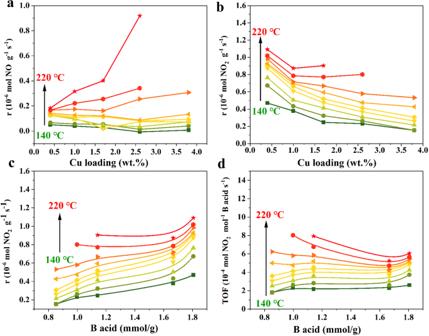Fig. 2: Kinetic analysis of fast SCR reaction. aNO reaction rates as a function of Cu loading over Cu-SSZ-13 catalysts in NO and NO2gas mixtures.bNO2reaction rates as a function of Cu loading over Cu-SSZ-13 in NO and NO2gas mixtures.cNO2reaction rates as a function of BASs over Cu-SSZ-13 in NO and NO2gas mixtures.dNO2turnover frequencies (TOFs) as a function of BASs in NO and NO2gas mixtures. The obtained Cu-SSZ-13 catalysts were Al-rich zeolites with Si/Al of ~5 and various Cu loadings from 0.4 to 3.8 wt.% (Supplementary Table 2 ). Catalyst evaluation The standard SCR (SSCR), fast SCR (FSCR) and slow SCR (NO 2 -SCR) reactions were carried out in a fixed-bed flow reactor system with an online Nicolet Is50 spectrometer, which was used to detect the concentrations of reactants and products. The SSCR conditions included 500 ppm NO and 500 ppm NH 3 ; the FSCR conditions included 250 ppm NO, 250 ppm NO 2 and 500 ppm NH 3 ; the NO 2 -SCR conditions included 300 ppm NO 2 and 500 ppm NH 3 . All the conditions included 3.5% H 2 O, 5%O 2 and N 2 balance. The total flow rate was 500 mL/min. The NO x (NO and NO 2 ) conversion was calculated at steady state: 
    NO conversion=(1-[NO]_out/[NO]_in)× 100%
 (5) 
    NO_2 conversion=(1-[NO_2]_out/[NO_2]_in)× 100%
 (6) 
    NO_x conversion=(1-[NO]_out+[NO_2]_out/[NO]_in+[NO_2]_in)× 100%
 (7) To conduct the kinetic studies, the gas hourly space velocity (GHSV) was controlled by adjusting the catalyst weight. The GHSV of SSCR, FSCR and NO 2 -SCR were about ~800,000 h −1 , ~1,000,0000 h −1 and ~2,000,000 h −1 , respectively. The reaction rates (r) in this study were normalized by catalyst weight based on Eq. ( 8 ). 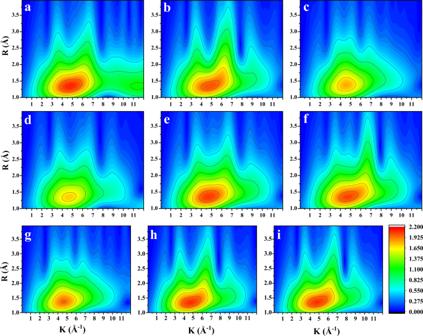Fig. 3: WT plots for EXAFS spectra of Cu-SSZ-13 treated under different conditions at 200 °C. aCu-SSZ-13 pretreated in O2/He.bNO adsorption.cNH3adsorption.dNO + NH3adsorption.eNO + NH3co-adsorption followed by reaction with O2.fNO + NH3co-adsorption followed by reaction with NO2.gSSCR conditions.hFSCR conditions.iNO2-SCR conditions. The activation energies (Ea) were calculated by the Arrhenius Eq. ( 9 ). r=F_NO_x∙X_NO_x/W_cat
 (8) 
    r=[NO_x]_0Ae^(-Ea/RT)
 (9) where F NOx represents the NO x flow rate (mol/s), X NOx represents the NO x conversion, W cat is the mass of the catalyst (g), and [NO x ] 0 is the inlet concentration of NO x . NOx represents NO, NO 2 or a mixture of both. Characterization The elemental composition of the catalysts was measured by inductively coupled plasma atomic emission spectroscopy (ICP-AES). N 2 adsorption-desorption analysis of the samples was conducted on a Micromeritics ASAP 2020 instrument. The acid site distribution and contents were measured by NH 3 temperature-programmed desorption (NH 3 -TPD) using the NH 3 -SCR activity measurement instrument described above. Samples of about 30 mg were used and pretreated in 10% O 2 /N 2 at 500 °C for 30 min before cooling down to 120 °C. Then, the gas was changed to 500 ppm NH 3 /N 2 for 60 min, followed by N 2 purging for 60 min. Finally, the temperature was raised to 700 °C at a rate of 10 °C/min. The in situ X-ray absorption fine structure (in situ XAFS) experiments were performed on the 1W1B beamline of Beijing Synchrotron Radiation Facility (BSRF). The absorption data from −200 eV to 800 eV of the Cu K-edge (8979 eV) were collected. The sample was first pretreated in O 2 /He at 500 °C for 30 min before decreasing the temperature to 200 °C, after which the Pre. spectra were collected. Then, the sample was exposed to 500 ppm NH 3 /He, 500 ppm NO/He and 500 ppm NH 3 /He + 500 ppm NO/He for 60 min, respectively, and spectra were collected. After reduction by (NO+NH 3 )/He, the sample was exposed to 5% O 2 /N 2 and 500 ppm NO 2 /N 2 for 60 min, respectively, to obtain the absorption data for the oxidized sample. Moreover, the in situ absorption data were collected after the pretreated samples were exposed to SSCR, FSCR and NO 2 -SCR atmospheres for 60 min. The X-ray absorption near-edge structure (XANES) data were background-corrected and normalized using the Athena module implemented in the IFFEFIT software package [44] . Extended X-ray absorption fine structure (EXAFS) data were analyzed and fitted using Athena and Artemis (3.0 < k < 13.0 Å −1 ). An amplitude reduction factor (S 0 2 ) of 0.85 was used for all the fitted data sets. Wavelet transform (WT) analysis of the EXAFS was performed to precisely investigate the local coordination environment of copper species. Computational details Spin-polarized periodic DFT calculations were carried out with the Vienna ab initio simulation package (VASP) [45] The Perdew−Burke−Ernzerhof (PBE) generalized gradient approximation was adopted with the van der Waals correction proposed by Grimme (i.e., DFT-D3 method) [46] . The Kohn-Sham orbitals were expanded with a plane-wave basis set with a cutoff energy of 500 eV, and the plane augmented wave (PAW) method was used to describe the interaction between the valence electrons and the cores [47] . The DFT + U method was applied to Cu 3d states with U eff = 6.0 eV to describe the on-site Coulomb interactions [29] , [48] . During geometrical optimization, the self-consistent-field electronic energies were converged to 1 × 10 −5 eV and all other atoms were fully relaxed until the maximum force on the atoms was less than 2 × 10 −2 eV/Å. The Brillouin zone was sampled with a Monkhorst-Pack k-point grid of 1 × 2 × 2. The Gaussian smearing method was utilized, with a smearing width of 0.2 eV. The transition states of elementary steps were located using the climbing image nudged elastic band (CI-NEB) method with several intermediate images between initial and final states [49] , [50] . Thermodynamic data were processed with the VASPKIT code [51] and the Gibbs free energies were calculated at 200 °C. The SSZ-13 zeolite structure was modelled using two rhombohedral unit cells (24 tetrahedrally coordinated atoms) with size of 18.84 Å × 9.42 Å × 9.42 Å (Supplementary Fig. 20 ). One Si atom was replaced by one Al atom in each double 6-membered ring, resulting in a model with a Si/Al ratio of 11. One H atom was introduced onto one of the O atoms connected with each Al atom to keep the structure charge-neutral. 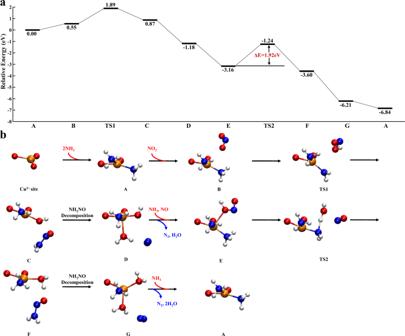Fig. 4: Reaction pathway of the fast SCR cycle at Z2CuIIsite. aGibbs free energy profile.bOptimized geometries of the reactants, transition states (TSs) and products for all elementary steps are presented in the lower panel. Except for the O atoms linked to the Cu2+ion, all other atoms of the zeolite framework are omitted for clarity. Orange, red, blue and white circles denote Cu, O, N and H atoms, respectively. 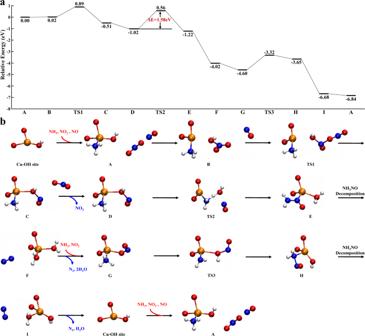Fig. 5: Reaction pathway of the fast SCR cycle at ZCuIIOH site. aGibbs free energy profile.bOptimized geometries of the reactants, TSs and products for all elementary steps are presented in the lower panel. Except for the two O atoms linked to the Cu-OH group, all other atoms of the zeolite framework are omitted for clarity. All legends are the same as those in Fig.4. 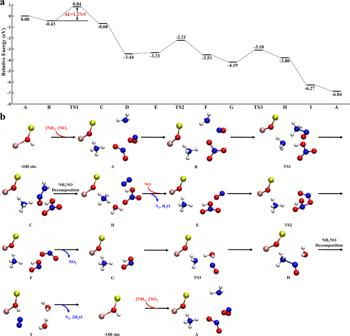Fig. 6: Reaction pathway of the fast SCR cycle at BAS. aGibbs free energy profile.bOptimized geometries of the reactants, TSs and products for all elementary steps. Except for the Si and Al atoms linked to the OH group, all other atoms of the zeolite framework are omitted for clarity. Yellow and pink circles denote Si and Al atoms, respectively. All other legends are the same as those in Fig.4. Based on previous studies [4] , [29] , the present computational settings and models were reliable for investigating the NH 3 -SCR mechanism over Cu-SSZ-13 zeolites.